An influenza virus-inspired polymer system for the timed release of siRNA Small interfering RNA silences specific genes by interfering with mRNA translation, and acts to modulate or inhibit specific biological pathways; a therapy that holds great promise in the cure of many diseases. However, the naked small interfering RNA is susceptible to degradation by plasma and tissue nucleases and due to its negative charge unable to cross the cell membrane. Here we report a new polymer carrier designed to mimic the influenza virus escape mechanism from the endosome, followed by a timed release of the small interfering RNA in the cytosol through a self-catalyzed polymer degradation process. Our polymer changes to a negatively charged and non-toxic polymer after the release of small interfering RNA, presenting potential for multiple repeat doses and long-term treatment of diseases. Small interfering RNA (siRNA) silences specific genes by interfering with mRNA translation, and therefore acts to modulate or inhibit specific biological pathways [1] , [2] , [3] . The siRNA-based therapy holds great promise in the cure of cancers and many other diseases. However, the naked siRNA is susceptible to degradation by plasma and tissue nucleases and is unable to cross the cell membrane due to its negative charge. This has necessitated the design of delivery vehicles to overcome the inherent siRNA cell transport barriers. Amongst many investigated approaches, the initial work with viral delivery carriers showed great promise for delivering DNA and other biomolecules [4] , [5] . Viruses have evolved with exquisite strategies to deliver their payload efficiently within a cell; for example, the enveloped influenza virus easily appropriates the cellular machinery to replicate itself [6] . This virus first becomes endocytosed, and utilizes this transportation process to reach the inner parts of the cell. Before reaching the lysosome, the acidic pH triggers a rapid geometric conformational change of the haemagglutinin (HA) protein, releasing the HA2 membrane fusion peptide that binds and facilitates fusion of the virus with the endosome membrane. The virus escapes into the cytosol where it then proceeds to replicate its genome [7] . However, despite the above advantages, viral delivery devices have associated safety concerns due to non-specific interruption of genes and induction of an immune response [4] , [5] . Development of non-viral siRNA delivery systems incorporating the strategies of the virus could provide a safer, cheaper and effective treatment for various diseases [8] , [9] . Among synthetic delivery vehicles, cationic polymers and lyposomes are widely known as nanocarriers for siRNA; they bind via electrostatic interactions to form complexes with the siRNA that are rapidly taken up by cells [10] , [11] . The polymer carriers usually incorporate a pH buffering molecule that acts as a ‘proton sponge’ or binds to the endosome membrane to facilitate their escape [12] , [13] . Although such systems have demonstrated utility in nonhuman primate studies for liver-related diseases due to the natural accumulation of the carrier in the liver [14] , [15] , [16] , [17] , the permanent cationic charge of the nanocarriers [18] , [19] makes release of the siRNA difficult [20] , [21] , [22] . The accumulation of cationic species could result in unwanted toxicity especially when administered in multiple doses. To overcome the release problem of siRNA, polymers have been designed to incorporate side chain molecules that trigger a release when stimulated using temperature [23] , pH [24] , redox potential [25] , [26] , light [27] , electrical pulse [28] , [29] and enzymatic degradation [30] , [31] . Such release mechanisms rely on either external (remote) or environmental stimuli. The complication arises in that many tissues and organs are not remotely accessible, and environmentally triggered stimuli can vary between cell lines and even within the same tissue or organ. Furthermore, after degradation, the polymers should form biologically benign particles avoiding toxic buildup in the tissues [32] , [33] . In the work reported here, we overcame these delivery challenges by designing our polymer carrier to deliver siRNA using some of the strategies inspired by viruses. The polymer carrier consists of a diblock copolymer with a first block of poly(2-dimethylaminoethyl acrylate) (PDMAEA, p K a~7.1). The PDMAEA block is cationic at physiological pH and degrades into the negatively charged and non-toxic poly(acrylic acid) (PAA) ( Fig. 1a ) in water through a self-catalyzed hydrolysis mechanism [32] . The degradation time to form PAA is independent of pH (as tested between pH 5.5 and 10.1) and the molecular weight of PDMAEA. This block segment can therefore bind strongly to siRNA and release it at a defined time (that is, ‘timed release’) independent of the physiological pH, allowing the delivery of siRNA into tissues not accessible through external or environmental triggers. The resulting negatively charged polymer should be relatively benign after release even after multiple doses. A second block consisting of P( N -(3-(1 H -imidazol-1-yl)propyl)acrylamide (PImPAA) and poly(butyl acrylate) (PBA) [18] was designed to induce fusion with the endosome membrane (and act in a similar way to the fusion peptide HA2) that results in escape of the polymer/siRNA complex to the cytosol where release of the siRNA can occur after degradation to PAA (see Fig. 1a ). In this work, we designed a range of block copolymers ( Fig. 1b ) to examine the mode of delivery and release using an osteosarcoma cell line as a proven siRNA model system, and determine cell death through siRNA knockdown of the polo-like kinase 1 (PLK1) pathway. The best polymer carrier from this study was then trialed in vitro to silence the MAPK–ERK1/2 pathway in primary chondrocytes. 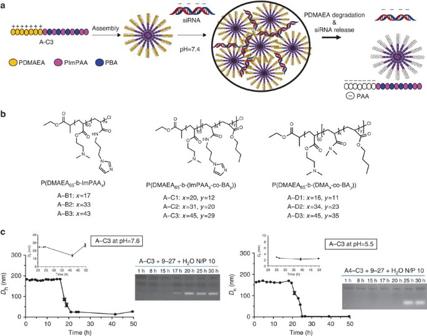Figure 1: Polymer structure and assembly. (a) Mechanism for polymer assembly, binding with siRNA and release of siRNA through a self-catalyzed degradation of PDMAEA, (b) chemical structures of the nine block copolymers, and (c) degradation profile of polymer A–C3 at pH 7.6 and 5.5 when complexes with oligo DNA as measured by DLS, and the time for release of the oligo DNA from the polymer carrier. Figure 1: Polymer structure and assembly. ( a ) Mechanism for polymer assembly, binding with siRNA and release of siRNA through a self-catalyzed degradation of PDMAEA, ( b ) chemical structures of the nine block copolymers, and ( c ) degradation profile of polymer A–C3 at pH 7.6 and 5.5 when complexes with oligo DNA as measured by DLS, and the time for release of the oligo DNA from the polymer carrier. Full size image Synthesis and physiochemical properties of polymers Single electron transfer-living radical polymerization (SET-LRP) [34] , [35] of DMAEA produced PDMAEA (polymer A in Supplementary Methods and Supplementary Table S1 in Supporting Information) with a number-average molecular weight ( M n ) of 4,200 and a polydispersity index (PDI) of 1.29 determined by size exclusion chromatography based on polystyrene standards and neglecting differences in polymer hydrodynamic volume (see Supplementary Figs S1–S3 ). A more accurate value of 9,430 determined by 1 H NMR showed that the polymer consisted of 65 DMAEA units. This polymer was previously tested as a delivery vehicle for siRNA, showing >90% cell uptake after 4 h and low cytotoxicity [32] , [33] , and thus was used as the first block in this work. PDMAEA 65 was extended with blocks containing units of ImPAA, BA and/or dimethylacrylamide (DMA) comonomers as shown in Fig. 1b using the SET-LRP technique. Conversion of monomer to polymer was kept low (<40%) to avoid high levels of radical–radical termination and further maintain a high -Cl chain-end functionality to produce block copolymers (A–B1 to A–D3) with PDIs below 1.3 ( Supplementary Table S1 ). The number of repeating units for all comonomers was given in Fig. 1b and Supplementary Table S1 based on 1 H NMR analysis (see Supplementary Figs S4–S7 ). Complexation of an oligo DNA (23 bp) with the A–B polymer series in water showed an increase in size (i.e. diameter, D h ) from ~5 to 200 nm with an increase in the N/P ratio (i.e. nitrogen to phosphorus ratio) from 0 to 10 (see Supplementary Table S2 ). A similar trend was found for the A–C and A–D series, but here the initial D h (at N/P=0) showed that the incorporation of the hydrophobic monomers, BA and ImPAA, in the second block gave small polymeric micelles of ~15 to 20 nm (A–C1 to A–C3). The A–C3 polymer candidate showed that at an N/P ratio of 10 at pH 7.6, these small 20 nm nanoparticles aggregated with the oligo DNA to result into a narrow particle size distribution close to 200 nm in size as shown in Fig. 1c . Leaving the complex of A–C3/oligo DNA in water at pH 7.6 resulted in its degradation after 17 h, whereby the size decreased from 200 to 20 nm and the oligo DNA was fully released (see the Agarose gel in Fig. 1c ). A similar profile was found when the complex was kept at pH 5.5, with full release of the oligo DNA after 25 h and a size decrease to 5 nm ( Fig. 1c ) corresponding to the size of an individual polymer coil (i.e. unimer) in solution. This result suggests that the siRNA (with a similar size to the oligo DNA) can still be complexed with the polymer in the low pH environment of the endosome, and if escape from the endosome is faster than the release time of ~17 h, the siRNA has a great chance of being released within the cytosol. The similar degradation profiles of A–C3 in pH 5.5 and 7.6 further supported a non-triggered and timed-release mechanism of the siRNA from the polymer carrier. In addition, the degradation profiles for A–B3 and A–D3 at pH 7.6 and 5.5 were all similar to A–C3, suggesting that only the degradation of PDMAEA to PAA plays the dominant role for release of oligo DNA (see Supplementary Figs S9–S14 ). In vitro RNAi-mediated knockdown of PLK1 in osteosarcoma Osteosarcoma is a bone cancer prevalent in young people, with poor survival rates. Polo-like kinase 1 (PLK1) has an important role in maintaining tumorgenic phenotype of osteosarcoma cells [36] . Its knockdown using siRNA delivery should induce selective growth arrest and cell death. In this work, we used the U-2OS cell line as an in vitro model system to test our polymers (from Fig. 1b ) for knockdown using a previously screened siRNA [36] . We evaluated the knockdown of U-2OS cells using our polymer-loaded siRNA complexes via a cell viability assay. Four siRNAs were used: (i) siRNA targeting PLK1, (ii) universal negative control (Mission siRNA, Sigma-Aldrich), (iii) scrambled siRNA for PLK, and (iv) a negative control S10 siRNA that targets another pathway [37] . The polymer-loaded siRNA complexes were also compared with oligofectamine/siRNA complexes, in which oligofectamine is regarded as the gold standard for siRNA delivery. Solutions of the polymer and siRNA in PBS buffer at various N/P ratios (that is, 0 to 10) were mixed and incubated for 30 min at room temperature. The complex was then added to the cells in complete DMEM media at 37 °C, and after 4 h, the cells were washed to remove any complex not taken up by the cells and incubated for another 48 h. The concentration of siRNA used in this assay was 50 nM. It can be seen that polymer A loaded with siRNA by itself (that is, PDMAEA 65 ) showed little toxicity and little or no knockdown compared with oligofectamine-loaded siRNA targeting PLK1 (see Supplementary Fig S15A ). Incorporating an ImPAA second block (A–B series) to act as either a proton sponge or fusogenic polymer also showed little toxicity and little or no cell death irrespective of the molecular weight of the second block when loaded with PLK1 siRNA( Fig. 2a and Supplementary Fig. S15B–D ). The results suggest that even with the inclusion of ImPAA (similar functional group to histidine), the polymer carrier could not escape the endosome. Polymer series A–C incorporating not only ImPAA but hydropobic BA was synthesized to further assist in endosome escape. The cell viability data ( Fig. 2b and Supplementary Fig. S16 ) using A–C2 and A–C3 loaded with PLK1 siRNA showed little or no cell death at N/P ratios below 10. At an N/P ratio of 10, both polymers loaded with PLK1 siRNA complexes showed excellent knockdown (>80%) and little toxicity. This amount of cell viability loss specific to targeting the PLK1 pathway was substantially better than oligofectamine/siRNA. To test whether cell death was due to the combination of ImPAA and BA in the second block or as a result of only BA, we synthesized the A–D polymer series consisting of BA and DMA in the second block. The results for A–D3 ( Fig. 2c ) and A–D1 and A–D2 ( Supplementary Fig. S17 ) showed that without ImPAA there was no observed cell death. The combination of ImPAA and BA in the second block demonstrates that both comonomers act synergistically to allow escape of the polymer/siRNA complex from the endosome into the cytosol, most probably due to the combined ionic and hydrophobic interactions with the endosome membrane. To confirm that cell death was primarily due to siRNA targeting PLK, we tested two different control siRNAs (universal negative control (denoted as Uni) and a scrambled siRNA (denoted as Scr)) delivered with polymer A–C3, and the data given in Fig. 2d shows that there is no knockdown with either of these siRNAs. Further, the cell viability of polymer A–C3 alone before ( Supplementary Fig. S19A ) and after ( Supplementary Fig. S19B ) degradation (that is, self-catalyze to poly(acrylic acid)) of the PDMAEA block in A–C3 showed little or no cell toxicity even at an NP ratio of 20. These results collectively demonstrate the excellent knockdown potential of A–C3 with little or no cytotoxicity. 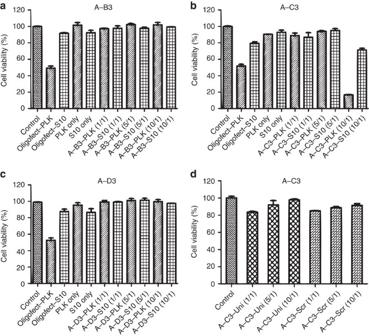Figure 2:In vitroknockdown efficiencies. U-2OS cellin vitroknockdown efficiency of (a) P(DMAEA65-b-ImPAA43) (A–B3), (b) P(DMAEA65-b-(ImPAA45-co-BA29)) (A–C3), and (c) P(DMAEA65-b-(DMA45-co-BA35)) (A–D3) complexes with siRNA targeting PLK and negative siRNA control S10 at N/P ratios of 1, 5 and 10 after 30 min complexation in water. The polymers were added to the cells and left to transfect for 4 h, and further incubated for 48 h. Controls used were untreated (Control), PLK/Oligofectamine complex (Oligofect–PLK), S10/Oligofectamine (Oligofect–S10) complexes, PLK siRNA only (PLK only) and S10 siRNA only (S10 only). Concentrations of PLK and S10 used was 50 nM. The data are reported as the mean±s.e.m. of three replicates. (d) U-2OS cell viability of P(DMAEA)65-P(ImPAA45-co-BA29) (A–C3) complexes with universal siRNA (Uni) and scrambled siRNA (Scr) at N/P ratio 1, 5 and 10 after 30 min complexation in water, 4 h transfection and 48 h incubation. Controls used are untreated (Control). Concentration of universal siRNA and scrambled siRNA used is 50 nM. The data are reported as the mean±standard error of the mean of two replicates. Values in parenthesis are N/P ratios. Figure 2: In vitro knockdown efficiencies. U-2OS cell in vitro knockdown efficiency of ( a ) P(DMAEA 65 -b-ImPAA 43 ) (A–B3), ( b ) P(DMAEA 65 -b-(ImPAA 45 -co-BA 29 )) (A–C3), and ( c ) P(DMAEA 65 -b-(DMA 45 -co-BA 35 )) (A–D3) complexes with siRNA targeting PLK and negative siRNA control S10 at N/P ratios of 1, 5 and 10 after 30 min complexation in water. The polymers were added to the cells and left to transfect for 4 h, and further incubated for 48 h. Controls used were untreated (Control), PLK/Oligofectamine complex (Oligofect–PLK), S10/Oligofectamine (Oligofect–S10) complexes, PLK siRNA only (PLK only) and S10 siRNA only (S10 only). Concentrations of PLK and S10 used was 50 nM. The data are reported as the mean±s.e.m. of three replicates. ( d ) U-2OS cell viability of P(DMAEA) 65 -P(ImPAA 45 -co-BA 29 ) (A–C3) complexes with universal siRNA (Uni) and scrambled siRNA (Scr) at N/P ratio 1, 5 and 10 after 30 min complexation in water, 4 h transfection and 48 h incubation. Controls used are untreated (Control). Concentration of universal siRNA and scrambled siRNA used is 50 nM. The data are reported as the mean±standard error of the mean of two replicates. Values in parenthesis are N/P ratios. Full size image Escape from the endosome is thus a key feature of our polymer carrier that allows effective delivery of the siRNA to the cytosol. Two mechanisms have been proposed for pH-responsive polymers (for example, with imidazole groups) to facilitate escape [12] , [13] : (i) an osmotic gradient caused by a flux of counter ions to maintain the ionic strength in the endosome and thus induce endosome lysis, or (ii) interaction of the imidazole groups with the endosome membrane. Our results showed that the siRNA targeting PLK gave ~80% knockdown with little or no toxicity from the polymer A–C3. The requirement for the combination of ImPAA and BA in the second block (A–C series) demonstrates the capability of these monomer units to fuse with the endosome membrane and facilitate escape. The ImPAA (that is, imidazole) side groups become highly protonated when the pH drops below its p K a of ~6, which should enable these positive charges to interact with the negatively charged endosome membrane and induce a bilayer phase separation. The BA monomer units should further interact with the membrane through hydrophobic interactions and facilitate fusion with the membrane leading to escape. As described earlier, the fusogenic second block in A–C2 and A–C3 is located in the core of the micelle with a size of ~20 nm ( Supplementary Table S2 ), and must therefore be exposed to the surface of the micelles when the pH drops in the endosome to interact with the endosome membrane, mimicking structural reorganization found for the influenza virus. When the polymer without siRNA was self-assembled in water at pH 7.6, small micelles formed with a size of ~20 nm ( Supplementary Table S3 ). When the pH was decreased to 5.5, the polymer was fully water soluble and the polymer chains dissociated from the micelle forming unimers of ~5 nm. Increasing the pH back to 7.6 resulted in reconstitution (self-assembly) of the unimers back to small ~20 nm particles. The polymer (A–C3)/oligo DNA complex showed no change in particle size when the pH was decreased from 7.6 to 5.5 ( Fig. 1 ). These results suggested that the 20 nm polymer particles when complex with the siRNA formed a large 200 nm aggregate, and when in the endosome, the size of the aggregate did not change due to the strong ionic binding between the siRNA and polymer chains even though the ImPAA groups were now cationic and hydrophilic. Our observations are consistent with the fully water soluble ImPAA and BA second block reorganizing in the endosome to be exposed to the exterior of the aggregate, allowing fusion and escape from the endosome membrane. Once in the cytosol, release of the siRNA occurs after 17 h, which acts to interfere with the specific mRNA. In vitro RNAi-mediated knockdown of ERK in osteoarthritis chrondrocytes The MAPK–ERK (mitogen activated protein kinase-extracellular signal-regulated kinase) cell signaling pathway has been identified as one of the central regulatory factors in osteoarthritis (OA) progression, especially in the altered communication between the osteoarthritic cartilage and the subchondral bone [38] . We evaluated the efficiency of the polymer A–C3 loaded with siRNA targeting ERK in OA chondrocytes. Articular cartilage cells (ACCs) were isolated from OA cartilage, and the early passage cells (P1-2) were used in the in vitro experiments. The polymer/siRNA concentrations used in this study showed no significant cytotoxic effects in siRNA treatment groups using the standard LDH (lactate dehydrogenase) assay ( Fig. 3a ). The A–C3 polymer loaded with ERK siRNA diminished ERK1/2 (ERK1/2) levels in severe OA ACCs measured using the western blot analysis after 48 h ( Fig. 3b ). This in vitro knockdown of ERK enhanced chondrocyte differentiation and impaired pathological phenotytic changes in severe OA ACCs ( Fig. 3c ). The polymer A–C3 alone was not toxic to the OA ACCs even at an NP ratio of 20 before ( Supplementary Fig. S20A ) and after ( Supplementary Fig. S20B ) degradation of the PDMAEA part of the polymer. Knockdown by siRNA specific to the ERK pathway was further demonstrated using a universal negative siRNA control and a scrambled siRNA, both of which showed no knockdown capability ( Supplementary Fig. S21 ). ACCs from severe OA knee cartilage (Mankin score ≥6) showed a poor capacity for chondrogenic differentiation with higher levels of hypertrophic and degenerative markers. When A–C3-loaded ERK siRNA was delivered to the severe OA ACCs, the degradative enzymes of ADAMTS5 (disintegrin and metalloproteinase with thrombospondin motifs 5), MMP-13 (matrix metalloproteinases 13) and pathological hypertrophic markers of type 10 collagen (COL10) and Runt-related transcription factor-2 (RUNX2) were significantly decreased. In contrast, we observed increased levels of chondrogenic markers COL2 and AGAN ( Fig. 3c ). These findings collectively indicated that ERK siRNA loaded into our polymer (A–C3) improved the chondrogenic differentiation and inhibited the pathological degradative and hypertrophic changes in OA ACCs. 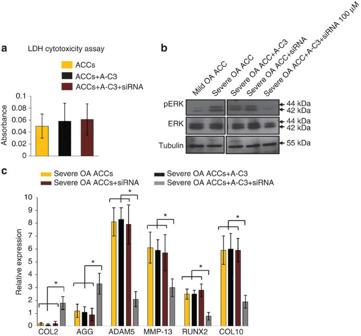Figure 3:In vitroeffects of ERK siRNA delivery on OA ACCs. (a) Cell cytotoxicity of ACCs treated with polymer and polymer+ERK siRNA after 48 h of transfection. Compared with control, there is no significant difference in cell cytotoxicity in either polymer or polymer+ERK siRNA group (P>0.05;n=5 in all instances). (b) Western blotting image showing the substantial downregulation of ERK in polymer+siRNA-treated severe OA ACCs. A representative bands obtained from three patients with similar results was shown. (c) qRT–PCR showed that chondrogenic markers such asCOL2andAGGwere upregulated and degradative and hypertrophic markers such as ADAMTS5, MMP-13 andCOL10were downregulated in severe OA ACCs treated with Polymer+ERK siRNA. mRNA levels were normalized against 18 S rRNA and the relative fold change gene expression is presented. Results are shown as mean±s.d. *P<0.05. Values are representative of five patients with similar results. Figure 3: In vitro effects of ERK siRNA delivery on OA ACCs. ( a ) Cell cytotoxicity of ACCs treated with polymer and polymer+ERK siRNA after 48 h of transfection. Compared with control, there is no significant difference in cell cytotoxicity in either polymer or polymer+ERK siRNA group ( P >0.05; n =5 in all instances). ( b ) Western blotting image showing the substantial downregulation of ERK in polymer+siRNA-treated severe OA ACCs. A representative bands obtained from three patients with similar results was shown. ( c ) qRT–PCR showed that chondrogenic markers such as COL2 and AGG were upregulated and degradative and hypertrophic markers such as ADAMTS5, MMP-13 and COL10 were downregulated in severe OA ACCs treated with Polymer+ERK siRNA. mRNA levels were normalized against 18 S rRNA and the relative fold change gene expression is presented. Results are shown as mean±s.d. * P <0.05. Values are representative of five patients with similar results. Full size image We demonstrate the use of a sophisticated polymer delivery carrier for the delivery of siRNA to silence distinct pathways. Our polymer was designed where one block binds electrostatically with siRNA and then degrades to a negatively charged side groups that repels and releases the siRNA. It takes 17 h in pH 7.6 to release the siRNA. This is more than sufficient time for the polymer carrier/siRNA to escape the endosome and release the siRNA in the cytosol. The second block consisting of ImPAA and BA resulted in a polymer carrier mimicking the escape mechanism of the influenza virus from the endosome into the cytosol. A distinct advantage of our polymer is that it forms a non-toxic negatively charged polymer, allowing the potential for multiple doses and effective treatment of the disease. Our polymer carrier was effective in siRNA knockdown with >80% of cell death when targeting the PLK1 pathway for osteosarcoma cancer cells, and when targeting the ERK1/2 pathway shown to be the key regulatory pathway in OA. These results demonstrate great promise for the application of our A–C3 polymer as an effective and safe siRNA delivery carrier for further applications in many diseases. Synthesis and characterization of polymers Details of the syntheses including materials used, and complete polymer characterization by size exclusion chromatography, 1 H nuclear magnetic resonance and dynamic light scattering and provided in the Supplementary Methods section, along with details of the agarose gel assays for binding and release studies. Osteocarcoma model assays Details of the osteocarcoma model assays, including in-vitro studies of knockdown of osteosarcoma U-2OS cells and examination of cell viability of osteosarcoma U-2OS cells using Cell Titer-Glo assay are provided in the Supplementary Methods section. Osteoarthritis model assays Details of the osteoarthritis model assays, including in-vitro cytotoxicity studies and examination of cell viability of osteosarcoma OA ACCs cells using Cell Titer-Glo assay are provided in the Supplementary Methods section. How to cite this article: Truong, N. P. et al . An influenza virus-inspired polymer system for the timed release of siRNA. Nat. Commun. 4:1902 doi: 10.1038/ncomms2905 (2013).